SHB1 and CCA1 interaction desensitizes light responses and enhances thermomorphogenesis Light and temperature are two important environmental signals to plants. After dawn, photo-activated phytochromes translocate into the nucleus and interact with a family of negative basic helix-loop-helix PIF regulators. Subsequent phosphorylation and degradation of PIFs triggers a series of photomorphogenic responses. However, excess light can damage the photosynthetic apparatus and leads to photoinhibition. Plants acclimate to a balanced state of photomorphogenesis to avoid photodamage. Here, we show that upregulation of PIF4 expression by SHB1 and CCA1 under red light represents a desensitization step. After dawn, the highly expressed circadian clock protein CCA1 brings circadian signals to the regulatory region of the PIF4 signaling hub. Recruitment of SHB1 by CCA1 modulates red light-specific induction of PIF4 expression thus integrating circadian and light signals. As noon approaches and light intensity and ambient temperature tend to increase, the SHB1–CCA1 interaction sustains PIF4 expression to trigger thermomorphogenic responses to changing light and temperature conditions. Light signal is an important abiotic environmental factor. The regulation of plant growth and development by light signals involves three major classes of photoreceptors, the red (R) and far-red (FR) light-absorbing phytochromes and the UV-A/blue light-absorbing cryptochromes and phototropins [1] . Arabidopsis thaliana has five phytochrome genes, PHYA to PHYE [2] , [3] , [4] . Phytochromes (phy) are photo-reversible between the red absorbing form (Pr) and the far-red absorbing form (Pfr). Following conversion to the biologically active Pfr form, phytochromes translocate into the nucleus and interact with an important subfamily of bHLH transcription factors, the phytochrome interacting factors (PIFs). Their interaction leads to their phosphorylation, ubiquitination, and degradation via the 26 S proteasome and alters gene expression rapidly [5] , [6] , [7] , [8] . PIFs play a variety of roles in regulating plant light responses, such as seed germination, seedling skotomorphogenesis, de-etiolation, shade avoidance, and flowering [9] , [10] , [11] . Photoreceptors and the circadian clock sense and integrate diurnal and seasonal changes in environmental signals and modulate plant growth and development. The circadian clock regulates adaptation of plants to the alternation of day and night. The initial model of the plant circadian clock is a feedback loop, including the central oscillator components circadian clock associated 1 (CCA1, an MYB transcription factor), late elongated hypocotyl (LHY, a homolog of CCA1), and timing of CAB2 expression 1 (TOC1) and its related pseudoresponse regulators (PRRs). CCA1 and LHY are the first two plant clock genes identified, and bind directly to the TOC1 promoter and repress TOC1 expression [12] , [13] , [14] , [15] . TOC1 is a DNA-binding transcriptional factor and functions as a general transcriptional repressor of clock genes including CCA1 and LHY [16] , [17] , [18] . Recently, a number of new components have been integrated into clock models. These include the reveille (RVE) family of MYB transcription factors, which act in a feedback loop as transcriptional activators [19] , [20] . In addition, light-regulated WD 1/2 (LWD1/2) and night light-inducible and clock-regulated 1/2 (LNK1/2) are also transcriptional activators involved in circadian clock function [21] , [22] . Light and temperature are the most dynamic parameters in plant growth and development. PIFs act as pivotal components in a cellular signaling hub integrating biotic and abiotic pathways to regulate plant growth [10] . For example, PIF4 mediates plant adaptation to elevated ambient temperature or thermomorphogenesis [23] , [24] . Developmental and morphological changes are induced by high ambient temperature below the heat stress range [25] . In Arabidopsis , the changes include increased elongation of hypocotyls and petioles, hyponastic growth, and development of thinner leaves [26] . In addition, pif4 exhibits an early flowering phenotype compared with wild type under high ambient temperature [23] . PIF4 coordinates this response by activating hormonal modules that subsequently regulate growth. PIF4 interacts with brassinazole-resistant 1 (BZR1), a transcription factor induced by brassinosteroid, and activates the expression of a number of downstream genes that drive shoot organ elongation [27] , [28] . PIF4 also directly regulates auxin levels by activating several auxin biosynthesis genes such as yucca 8 ( YUC8 ) to promote hypocotyl elongation and hyponastic leaf growth [29] , [30] . TOC1, the evening-expressed circadian clock protein, directly interacts with PIF4 and prevents its activation of downstream target genes, thereby suppressing thermomorphogenesis specifically at the end of day and evening [24] . Although light signals are fundamental to the growth and development of plants, excess light energy damages the photosynthetic apparatus and frequently enforces an inhibitory effect on photosynthesis known as photoinhibition [31] . Light inevitably generates excess reactive oxygen species (ROS) can be generated during photosynthesis under strong light, which can lead to photoinhibition and oxidative damage to the photosynthetic apparatus [32] , [33] , [34] , [35] . Photosynthetic organisms are able to acclimate to different environmental conditions to alleviate the detrimental effects of excess light on growth and viability [36] . For example, under excess light conditions, plants may acquire a balanced state of photomorphogenesis to avoid the absorption of excess light energy and to reduce photodamage through a feedback mechanism. Although the molecular mechanisms stimulating response to light are well established, those required for desensitization of perceived light signals remain less understood. SHB1 was initially isolated from the gain-of-function mutant short hypocotyl under blue 1 Dominant ( shb1-D ) based on its long hypocotyl phenotype under red, far-red, and blue light [37] . In shb1-D , a T-DNA is inserted 129 base pairs upstream of the SHB1 start codon and causes SHB1 overexpression. SHB1 contains an N-terminal SPX domain and a C-terminal EXS domain homologous to yeast suppressor of yeast GPA1 (SYG1) family proteins [37] . Its N terminus retains the function of full-length SHB1, and overaccumulation of the SHB1 C terminus causes a dominant-negative phenotype [38] . PIF4 expression is increased in shb1-D compared with wild type and decreased in shb1 partial loss-of-function mutant specifically under red light [37] . The molecular mechanism by which SHB1 regulates PIF4 expression specifically under red light and its biological implication are still unknown. In this study, SHB1 hijacks the highly expressed central oscillator component CCA1 and LHY in the morning and is targeted to the PIF4 promoter. During the day when light intensity and temperature increase, the SHB1–CCA1/LHY interaction sustains PIF4 expression in response to both red light and higher ambient temperature. This mechanism serves two important purposes: upregulate PIF4 expression to desensitize light responses for optimal photomorphogenesis, and enhance plant thermomorphogenesis for better survival under elevated ambient temperature. SHB1, CCA1, and LHY regulate PIF4 expression under red light In an early study, SHB1 specifically upregulated PIF4 expression under red light as assessed by real-time quantitative PCR and RNA gel blot hybridization analysis [37] . In general, PIF4 expression was induced by red light, downregulated in shb1 and upregulated in shb1-D compared with wild type under red light (Fig. 1a ). Although PIF1 , PIF3 , PIF5 , and PIF7 expression was induced by red light, only the red light-induced expression of PIF7 was partially compromised in shb1 but not in shb1-D (Supplementary Fig. 1a ). The rhythmic expression of PIF4 is controlled by the circadian clock [39] , [40] , [41] . We also examined the rhythmic expression of PIF4 in Col, shb1 , Ws, and shb1-D seedlings under continuous red light after growth under 12-hr dark and 12-hr 2 μmol m −2 s −1 red light for 7 days (Fig. 1b, c ). Samples were obtained at ZT0 and every 3 h thereafter for 36 h. Both shb1 and shb1-D mutations affected the magnitude but not the rhythmic pattern of PIF4 expression. Fig. 1 SHB1 and CCA1/LHY regulate PIF4 expression under red light. a PIF4 expression in 4-day-old Col, shb1 , Ws, and shb1-D seedlings in the dark and under 15 μmol  m −2 s −1 red light for 3 hr. * and ** indicate significance levels p < 0.05 and p < 0.01, respectively. ns indicates not significant by Student’s two-tailed heteroscedastic t tests in this figure and subsequent figures. PIF4 expression in Col and shb1 b or Ws and shb1-D c under continuous red light after entrained under 12-hr light and 12-hr dark for 7 days from two biological replicates. d PIF4 protein accumulation in Col, shb1 , Ws, and shb1-D under 12-hr red light and 12-hr dark photoperiod, shown as representative images from three biological replicates. e PIF4 protein quantification normalized to actin with standard error bars. The control blot shows PIF4 accumulation in Ws, shb1-D and pif4 at ZT6. f PIF4 expression in Ws, cca1, lhy, and cca1 lhy in the dark and under 15 μmol m −2 s −1 red light. Expression of PIF4 in each sample was normalized to that of UBQ10 , and data are presented as the means ± SE. Source data are provided as a Source Data file Full size image When PIF4 was driven by its native promoter, PIF4 protein accumulation correlated with PIF4 transcription, and PIF4 protein accumulated during the light period from ZT0 to ZT8 but not in the dark period from ZT12 to ZT20 under short days (8 h white light/16 h dark) [42] . Under a 12-hr red light and 12-hr dark photoperiod, PIF4 protein was detectable after ZT3 and reached its peak accumulation at ZT9, correlating well with PIF4 mRNA level (Fig. 1b–e ). Before ZT3, the lower level of PIF4 accumulation was probably due to the low level of PIF4 mRNA and/or PIF4 degradation after the initial illumination with red light. PIF4 accumulation was strongly enhanced in shb1-D from ZT6 to ZT12 but moderately reduced in shb1 from ZT6 to ZT12 and beyond (Fig. 1e ). SHB1 is unable to target to the PIF4 locus given that it contains no recognizable DNA-binding domain. Other transcription factors likely recruit SHB1 to the PIF4 promoter. We identified several potential MYB-binding elements ATATC(T/A) in the PIF4 promoter ( http://meme-suite.org/ ). In Arabidopsis , MYB family transcription factors have multiple functions [43] . The two central circadian clock components, CCA1 and LHY, are potential candidates. PIF4 expression was reduced in the cca1 or the lhy single mutant, and was further reduced in the cca1 lhy double mutant (Fig. 1f ). PIF4 expression was not altered in cca1 or lhy single mutants or in the cca1 lhy double mutant in the dark. The rhythmic expression of PIF4 is controlled by the circadian clock [39] , [40] , [41] . In the cca1 lhy double mutant, the rhythmic expression of PIF4 was completely compromised (Supplementary Fig. 1b ). In addition, SHB1 expression was not rhythmically expressed compared with CCA1 and LHY (Supplementary Fig. 1c ). Therefore, CCA1 and LHY are required for the rhythmic expression of PIF4 , and SHB1 enhances but does not alter the pattern of PIF4 rhythmic expression. Genetic interaction between PIF4 and SHB1 , CCA1, and LHY We investigated the genetic interaction between SHB1 and PIF4 by measuring the hypocotyl elongation of Ws, pif4 , shb1-D and the shb1-D pif4 double mutant under red light. shb1-D exhibited a long hypocotyl, and pif4 exhibited a short hypocotyl compared with wild type. The shb1-D pif4 double mutant exhibited a slightly longer hypocotyl compared with pif4 , but it was considerably much shorter than that of shb1-D (Fig. 2a ). The shb1-D mutation still increased hypocotyl length in the pif4 mutant background or SHB1 also promoted hypocotyl elongation independent of PIF4, SHB1 may target to other genes in addition to PIF4 to influence hypocotyl elongation. Fig. 2 Genetic interaction of PIF4 with SHB1 or CCA1/LHY . Hypocotyl lengths of Ws, pif4 , shb1-D, and shb1-D pif4 a ; Ws, cca1 , lhy, and cca1 lhy b ; three 35 S::PIF4:GFP ( pMDC83 ) transgenic lines in Ws or cca1 lhy c ; and Ws, shb1-D, cca1 lhy, and shb1-D cca1 lhy d in the dark or under 10 μmol m −2 s −1 red light for 4 days. Bar = 5 mm. Box plots display medians as horizontal lines, interquartile ranges as boxes and whiskers extending 1.5 times the interquartile range in this and subsequent figures. Significance levels by Student’s two-tailed heteroscedastic t tests in a: p < 0.001 between a and b , a and c , a and d , b and d , or c and d ; in b : p < 0.01 between a and b , p < 0.001 between a and c or b and c ; in c : p < 0.001 between a and b or c and d ; in d : p < 0.001 between a and b , a and c or b and c . e PIF4 expression in Ws, shb1-D, cca1 lhy, and shb1-D cca1 lhy . PIF4 expression in each sample was normalized to that of UBQ10 , and data are presented as the means ± SE. Source data are provided as a Source Data file Full size image Although CCA1 and LHY are redundant genes, the cca1 or lhy single mutant exhibited a short hypocotyl similar to that of pif4 , and the cca1 lhy double mutant exhibited a considerably shorter hypocotyl compared with each single cca1 or lhy mutant (Fig. 2b ). To study their epistasis, we overexpressed PIF4:GFP driven by the CaMV 35 S promoter in Ws and crossed three independent transgenes to the cca1 lhy background (Supplementary Fig. 2a ). The hypocotyl of the 35 S :: PIF4 : GFP transgenic lines was considerably elongated in Ws (Fig. 2c ). Overexpression of PIF4::GFP in cca1 lhy generated a shorter hypocotyl compared with that in Ws, but a considerably longer hypocotyl compared with the cca1 lhy double mutant. Combining the results demonstrating that the red light-induced PIF4 expression relies on CCA1 and LHY (Fig. 1f and Supplementary Fig. 1b ), we conclude that PIF4 acts downstream of CCA1 and LHY. The shb1 mutation caused a minimal hypocotyl phenotype but affected PIF4 expression under red light [37] . The shb1 mutant allele also showed a partial loss-of-function phenotype in endosperm proliferation and cellularization [44] , [45] . Triple shb1 cca1 lhy mutant was constructed, and the hypocotyl length and PIF4 expression were barely affected when shb1 was introduced to cca1 lhy (Supplementary Fig. 2b, c ). In shb1 , a T-DNA is inserted at the 8th intron of the SHB1 gene (SALK_128406), and a truncated message was still produced (Supplementary Fig. 2d, e ). Given the extremely low level of SHB1 expression and the low sensitivity of Taq polymerase used for semi-quantitative PCR analysis, we previously failed to detect the truncated message [37] . The full-length SHB1 protein contains 745 amino acids, and shb1 lacks the C-terminal 223 amino acids but retains the N-terminal 522 amino acids. Given that the N terminus of SHB1 is important for its function [38] , the truncated SHB1 in shb1 is partially functional. In contrast, a shb1-D cca1 lhy triple mutant showed a hypocotyl phenotype and PIF4 expression similar to that of the cca1 lhy double mutant (Fig. 2d, e and Supplementary Fig. 2f ). We examined the expression of SHB1 in shb1-D and shb1-D cca1 lhy triple mutant (Supplementary Fig. 2g ). The levels of SHB1 transcripts are comparable in shb1-D and shb1-D cca1 lhy . Thus, the promotion of hypocotyl and PIF4 expression by SHB1 under red light critically relies on CCA1 and LHY. Regulation of PIF4 expression enhances thermomorphogenesis Given that PIF4 is required for thermomorphogenesis, the induction of PIF4 expression by SHB1 and CCA1 may affect plant thermomorphogenesis. We examined hypocotyl growth responses of Ws, shb1 , pif4 , shb1-D, and the shb1-D pif4 double mutant to warm temperatures. Col or Ws showed a clear thermos-response and this response was slightly reduced in shb1 but almost disappeared in pif4 (Fig. 3a ). shb1-D enhanced the thermos-response with an elongated hypocotyl, and this enhancement was not completely blocked in shb1-D pif4 double mutant. Therefore, the thermo-induced hypocotyl elongation through PIF4 under higher temperature may not be entirely dependent on SHB1. Fig. 3 CCA1/LHY and SHB1 enhance PIF4 expression and thermomorphogenesis. Hypocotyl lengths of Col, shb1 , Ws, pif4 , shb1-D , and shb1-D pif4 a ; Ws, cca1 , lhy , and cca1 lhy b ; three 35 S::PIF4:GFP lines in Ws or cca1 lhy c ; and Ws, shb1-D , cca1 lhy, and shb1-D cca1 lhy d , e under 30 μmol m −2 s −1 white light at 20 °C for 7 days or 20 °C for 4 days followed by 29 °C for 3 days. Bar = 5 mm. Significance levels by Student’s two-tailed heteroscedastic t tests in a: p < 0.001 between a and b , c and d , c and e , c and f , d and e , or e and f and p < 0.01 between d and f ; in b : p < 0.001 between a and b ; in c : p < 0.001 between a and b or c and d ; in d : p < 0.001 between a and b , a and c or b and c . f PIF4 expression in Col , shb1 , Ws, shb1-D , cca1 lhy, and shb1-D cca1 lhy . Seedlings were grown at 20 °C for 5 days and then incubated at 20 °C or 29 °C for 4 h. PIF4 expression in each sample was normalized to that of UBQ10 , and data are presented as the means ± SE. Source data are provided as a Source Data file Full size image Furthermore, warm temperature-induced hypocotyl growth of either cca1 or lhy was similar to that of Ws, and cca1 lhy double mutations indeed reduced plant responses to warm temperatures (Fig. 3b ). Overexpression of PIF4 driven by the 35 S promoter enhanced the thermo-response in either Ws wild type or cca1 lhy backgrounds (Fig. 3c and Supplementary Fig. 3 ). PIF4-overexpression plants grown at 20 o C exhibited a longer hypocotyl and increasing the temperature to 29 o C caused a further elongation of the hypocotyl. However, the ratio of hypocotyl length at 20 o C versus 29 o C in PIF4 -overexpression plants was comparable in either a wild type or cca1 lhy double mutant background. Warm temperature-induced PIF4 expression was reduced in shb1 and cca1 lhy , but significantly enhanced in shb1-D compared with that in Col or Ws wild type (Fig. 3f ). Hypocotyls of the cca1 lhy double mutant were elongated in response to high temperature, and PIF4 expression was still upregulated under high temperatures in cca1 lhy . The degree of upregulation was comparable between the wild type and the mutants. Therefore, the induction of the PIF4-mediated thermos-response under high temperature may not completely rely on CCA1 and LHY. In general, SHB1 and CCA1/LHY may not be required for thermos-activation of PIF4, but the overall increase in PIF4 transcription increases the magnitude of the thermo-response. Both hypocotyl and PIF4 expression at 29 °C in shb1-D cca1 lhy triple mutant were higher than that of cca1 lhy double mutant, but lower than that of shb1-D (Fig. 3d–f ). In addition to CCA1/LHY, other transcription factors may participate in SHB1-meditated thermos-responses. SHB1, CCA1, and LHY associate with the PIF4 promoter We assessed whether SHB1 directly regulates PIF4 expression although SHB1 does not contain a recognizable DNA-binding motif. We performed ChIP experiments with a SHB1:GFP transgene driven by the 35 S promoter and anti-GFP antibody followed by quantitative PCR (qPCR) analysis. We used four pairs of primers that detect different regions in the PIF4 promoter (Fig. 4a ). The samples were collected at ZT3 (8 am as ZT0) for dark-grown plants without or with 3 h of red light treatment. SHB1 was associated with 4–3 fragment in the PIF4 promoter (Fig. 4b ). Slight enrichment was observed for the 4–4 genomic fragment but the results were not statistically significant. The SHB1:GFP construct caused a longer hypocotyl phenotype and elevated PIF4 expression (Supplementary Fig. 4a, b ). Fig. 4 SHB1 and CCA1/LHY are associated with the PIF4 promoter. a PIF4 promoter demonstrating the chromatin regions (4–1, 4–2, 4–3, and 4–4) used for ChIP-quantitative PCR analysis and the potential Myb-binding sites M1 and M2 (asterisks). Association of SHB1:GFP b and CCA1:FLAG or SHB1:GFP in cca1 lhy c with the PIF4 promoter. d Rhythmic association of CCA1, LHY, or SHB1:GFP with the PIF4 promoter under 12-hr dark and 12-hr red light cycles from two biological replicates. Enrichment of DNA fragments was quantified by qPCR and normalized to that of UBQ10 . e Rhythmic PIF4 expression at various ZT points in Ws and 35 S::SHB1:GFP transgenic plants under 12-hr dark and 12-hr red light cycles. Data are presented as the means ± SE calculated from two biological replicates. Source data are provided as a Source Data file Full size image Two MYB-binding sites, M1 and M2, were identified in these two fragments (Fig. 4a ). MYB transcription factors CCA1 or LHY may mediate the association of between SHB1 and the PIF4 promoter. We performed ChIP experiments with CCA1:FLAG and LHY:MYC transgenes driven by the 35 S promoter and anti-FLAG or anti-MYC antibodies, respectively. CCA1 and LHY were also associated with the PIF4 promoter, and the 4–3 fragment was enriched under red light (Fig. 4c and Supplementary Fig. 4c ). We further examined whether SHB1 remained associated with the PIF4 promoter if CCA1 and LHY are mutated. SHB1 was unable to associate with the 4–3 genomic fragment in the PIF4 promoter in cca1 lhy (Fig. 4c ). We examined the accumulation of SHB1:GFP in Ws and cca1 lhy , and their levels were comparable in either Ws or cca1 lhy in the dark and under red light at the time points sampled for ChIP analysis (Supplementary Fig. 4d ). SHB1:GFP overexpression caused a longer hypocotyl phenotype and elevated PIF4 expression under red light in Ws but not in cca1 lhy (Supplementary Fig. 4e, f ). CCA1:FLAG and LHY:MYC did not associated with the PIF4 promoter in the dark (Fig. 4c and Supplementary Fig. 4c ). CCA1:FLAG or LHY:MYC levels were comparable in the dark and under red light for 3 h when we sampled for ChIP analysis (Supplementary Fig. 4d ). LUX, a component of the evening complex (EC), recognizes a consensus element GATWCG and two different types of degenerate elements, GATWYG or GATWCK [46] . The 4–4 fragment has one consensus element GATTCG that is 210 bp from the CCA1/LHY-binding element in the PIF4 promoter. The 4–3 fragment contains one degenerate element, GATTCC, which is 90 bp away from the CCA1/LHY-binding element. In addition, another degenerate element, GATTTG, is 1 bp away from the forward primer of the 4–3 fragment. In the EC complex, LUX interacts with ELF3 and ELF3 interacts with ELF4. ELF4:GFP was associated with both 4–3 ( p < 0.018) and 4–4 ( p < 0.013) fragments in the dark, but less efficiently with the 4–4 ( p < 0.045) fragment under red light (Supplementary Fig. 5a ). ELF4:GFP accumulated at comparable levels in the dark and under red light (Supplementary Fig. 5b ). Through ChIP-quantitative PCR assays and genome-wide expression profiling, PRR5, PRR7, and PRR9 also bind to the upstream regions of PIF4 and other key transcription factor genes, and repress their expression [47] . We hypothesize that the occupation of the PIF4 promoter by the entire EC complex and/or the PRR proteins in the dark may interfere with the binding of CCA1 or LHY to the PIF4 promoter. To correlate SHB1 binding to the PIF4 promoter with the regulation of PIF4 expression, we performed rhythmic ChIP assay for CCA1, LHY, and SHB1 (Fig. 4d ). We used wild-type plants with antibodies against CCA1 or LHY and 35 S::SHB1:GFP transgenic plants. We used the 35 S promoter to drive SHB1 expression given that SHB1 native promoter is very weak and SHB1 expression is not rhythmic. The plants were grown under 12-hr red light and 12-hr dark and were sampled at ZT0 and every 3 h thereafter for 24 h. CCA1, LHY, and SHB1 were associated with the PIF4 promoter from ZT0 to ZT9 but not thereafter (Fig. 4d ). The ChIP peak at ZT9 coincided with a maximum level of PIF4 expression, and PIF4 mRNA levels declined after ZT9 (Fig. 4e ). Surprisingly, the CCA1 ChIP peak did not coincide with the CCA1 mRNA peak (Supplementary Fig. 1c and Fig. 4d ). There might be a gradual departure of the EC complex or PRRs. Alternatively, CCA1 and LHY proteins or the SHB1–CCA1/LHY complex is very stable under red light. As shown in an early study, a large number of CCA1 target genes of CCA exhibit a peak expression from ZT5 to ZT16 in LD diel conditions or LL constant light [48] . Among them, ERD7 has a similar expression pattern as PIF4 . Therefore, CCA1 plays a potentially large role in the regulation of morning-expressed genes. CCA1 and LHY bind the MYB element in the PIF4 promoter We identified two MYB-binding elements, M1 and M2, in the PIF4 promoter (Fig. 5a and Supplementary Fig. 6a ). In a yeast one-hybrid (Y1H) assay, CCA1 and LHY bound to a DNA fragment that contains both M1 and M2 MYB binding elements in the PIF4 promoter (Fig. 5b ). We then tested which MYB-binding element is recognized by CCA1 or LHY using a trimeric M1 or M2 element in tandem repeats (Fig. 5c and Supplementary Fig. 6b ). CCA1 and LHY bound to the trimeric M1 element but not the trimeric M2 element. We subsequently mutated the M1 element or M2 element by changing two conserved bases and assessed whether CCA1 or LHY recognizes the mutated element (Fig. 5c and Supplementary Fig. 6b ). Neither CCA1 nor LHY bound to the mutated trimeric M1 element. Fig. 5 CCA1 and LHY recognize MYB M1 box in the PIF4 promoter. a Potential MYB-binding element M1 is noted in red, and the bases mutated are noted in blue. mb and md indicate mutation by base substitution and deletion, respectively. Yeast one-hybrid assays for CCA1 or LHY in pGADT7 over a 424-bp fragment that contains both M1 and M2 elements from the PIF4 promoter in the pAbAi vector b and for CCA1 or LHY in pGADT7 over trimeric repeats of wild type (upper) or mutated (lower) M1 element c . Golden Y1H cells were grown on SD/-Leu/-Ura media with or without 300 ng/ml Aureobasidin A (AbA) selection. Hypocotyl lengths of Ws, pif4 and pPIF4 or pPIF4md :: PIF4 in pif4 d and Ws, shb1-D pif4 and pPIF4 or pPIF4md :: PIF4 in shb1-D pif4 e . PIF4 expression in Ws, pif4 and pPIF4 or pPIF4md :: PIF4 in pif4 f and Ws, shb1-D pif4 and pPIF4 or pPIF4md :: PIF4 in shb1-D pif4 g . The seedlings were grown in the dark or under 10 μmol m −2 s −1 red light for 4 days. Hypocotyl lengths of Ws, pif4 and pPIF4 or pPIF4md :: PIF4 in pif4 h and Ws, shb1-D pif4 and pPIF4 or pPIF4md :: PIF4 in shb1-D pif4 i under 30 μmol m −2 s −1 white light at 20 °C for 7 days or 20 °C for 4 days followed by 29 °C for 3 days. PIF4 expression in Ws, pif4 and pPIF4 or pPIF4md :: PIF4 in pif4 j and Ws, shb1-D pif4 and pPIF4 or pPIF4md :: PIF4 in shb1-D pif4 k grown at 20 °C for 5 days and then incubated at 20 °C or 29 °C for 4 h. Significance levels by Student’s two-tailed heteroscedastic t tests in d : p < 0.001 between a and b , p < 0.01 between a and c , p < 0.05 between b and c ; in e : p < 0.001 between a and b , a and c , b and c or c and d , p < 0.01 between a and d , p < 0.05 between b and d ; in h : p < 0.001 between a and b or b and c , p < 0.01 between a and c ; in i : p < 0.001 between a and b , a and c or b and c . Source data are provided as a Source Data file Full size image PIF4 gene driven by a PIF4 promoter that bears either a wide type or a deleted M1 box was subsequently introduced into pif4 or shb1-D pif4 background (Fig. 5a ). Three lines in each category with comparable transgene expression was examined for light- and thermo-responses (Supplementary Fig. 7a, b ). The pPIF4 :: PIF4 cassette with a deleted M1 box hardly rescued the pif4 hypocotyl phenotype in either pif4 or shb1-D pif4 background compared with that with a wild-type M1 box (Fig. 5d, e and Supplementary Fig. 7c, d ). Deletion of the M1 box completely abolished the red light-induced PIF4 expression (Fig. 5f, g ). Given the effect of M1 box deletion on pif4 hypocotyl phenotype was less-dramatic than that on PIF4 expression, other signaling pathways may be operated to compensate for the lack of PIF4-mediated hypocotyl elongation in those pPIF4md :: PIF4 lines. Delivery of the wild-type pPIF4 :: PIF4 cassette to pif4 rescued pif4 hypocotyl thermo-response (Fig. 5h, i and Supplementary Fig. 7e, f ). The pPIF4 :: PIF4 cassette with a deleted M1 box in either pif4 or shb1-D pif4 showed a considerable defect in rescuing pif4 hypocotyl thermo-response but less-dramatic compared with red light-mediated hypocotyl elongation (Fig. 5h, i and Supplementary Fig. 7e, f ). The same cassette with a deleted M1 box in either pif4 or shb1-D pif4 also reduced the magnitude of thermo-induced PIF4 expression but did not alter the thermo-induction pattern compared with the wild type cassette (Fig. 5j, k ). Therefore, regulated PIF4 expression by SHB1–CCA1/LHY only contributes partially to PIF4-mediated thermo-responses. Either CCA1 or LHY did not bind in vivo the PIF4 promoter with a deleted M1 box but showed certain affinity toward the base-substituted M1 box (Supplementary Fig. 7g and Supplementary Fig. 8a ). In contrast to the in vivo ChIP assays, the Y1H assays may mask the weak affinity of CCA1 or LHY toward the base-substituted M1 box since 300 ng/ml AbA was added in order to titrate off the background growth (Fig. 5b, c ). As the base-substituted M1 box was still partially active in vivo, the disruption of the PIF4-mediated light- and thermo-responses by base substitution was less dramatic compared with M1 box deletion (Supplementary Fig. 7g and Supplementary Fig. 8a–j ). CCA1 and LHY interact with SHB1 SHB1 and CCA1 or LHY were associated with the PIF4 promoter, and CCA1 and LHY were required for the association of SHB1 with the PIF4 promoter. We performed bimolecular fluorescence complementation (BiFC) assays in N. benthamiana leaves to test whether SHB1 physically interacts with CCA1 or LHY (Fig. 6a, b ). In this system, CCA1 or LHY was fused with YFP N , and SHB1 was fused with YFP C . All constructs were driven by the CaMV 35 S promoter. As controls, CCA1:YFP N or LHY:YFP N did not form a fluorescence pair with YFP C , and SHB1:YFP C did not form a fluorescence pair with YFP N (Fig. 6a ). Both CCA1:YFP N and LHY:YFP N interacted with SHB1:YFP C as shown in fluorescence images. We also presented confocal images for the interaction between CCA1:YFP N or LHY:YFP N and SHB1:YFP C (Fig. 6b ). Fig. 6 SHB1 co-acts with CCA1 and LHY. a BiFC fluorescent images of YFP N with SHB1:YFP C , CCA1:YFP N or LHY:YFP N with YFP C , and CCA1:YFP N or LHY:YFP N with SHB1:YFP C . b BiFC confocal images of CCA1:YFP N or LHY:YFP N with SHB1:YFP C . Images were captured 48–72 h in Nicotiana leaf epidermal cells after Agrobacteria transfection. Bar = 10 μm. c Co-immunoprecipitation (Co-IP) of CCA1:FLAG or LHY:MYC by SHB1:GFP in protein extracts prepared from transgenic Arabidopsis with anti-GFP antibody. d Effector, reporter, and reference constructs used. Arrowheads indicate transcription start sites, and NOS-T represents polyadenylation signal from the nopaline synthase gene. Asterisk indicates the location of the M1 element in the PIF4 promoter. Relative LUC/REN activity in cca1 lhy transformed with a reporter along with pCCA1::CCA1:MYC , pLHY::LHY:MYC or 35 S::SHB1:MYC e and in Col or phyB-9 transformed with reporter in the absence or presence of 35 S::SHB1:MYC f in the dark or under red light. Source data are provided as a Source Data file. g A model explaining the regulation of CCA1 or LHY and SHB1 over PIF4 expression. PIF4 expression is repressed by the evening complex (EC) or PRRs at early evening. Toward the end of night and after dawn, CCA1 recruits SHB1 to mediate red light induction of PIF4 expression. This constitutes a signaling loop to optimize photomorphogenesis and enhance thermomorphogenesis Full size image We next performed co-immunoprecipitation (co-IP) assays with protein extracts prepared from 35 S::SHB1:GFP and 35 S::CCA1:FLAG or 35 S::LHY:MYC transgenic Arabidopsis plants (Fig. 6c ). SHB1:GFP coprecipitated CCA1:FLAG or LHY:MYC, further confirming their direct physical interaction. The additional bands recognized by anti-GFP antibodies in the SHB1:GFP lane may represent degradation products of full-length SHB1:GFP (Source Data file). We also detected SHB1 interaction with either CCA1 or LHY by BiFC assays in the dark; however, the interaction occurred less frequently (Supplementary Fig. 9a ). We performed Co-IP experiments with the 35 S::SHB1:GFP transgenic plants in the dark and under red light, and detected CCA1 or LHY using anti-CCA1 or anti-LHY antibodies (Supplementary Fig. 9b ). Equal amounts of CCA1 or LHY were precipitated by SHB1:GFP in the dark and under red light. SHB1 N terminus interacts with the CCA1 or LHY C terminus SHB1 contains an N-terminal SPX domain and a C-terminal EXS domain [38] . The SPX domain retains the function of full-length SHB1, whereas the function of the EXS domain remains unknown. SHB1 localizes to the nucleus, and the EXS domain in SHB1 may exhibit a function distinct from those in other SYG1-like proteins. To map the interaction domain of SHB1 with CCA1 or LHY, we split SHB1 into the SHB1 N terminus (N520) that contains 520 amino acids and the putative SPX domain and the SHB1 C terminus (C325) that contains 325 amino acids and the EXS domain (Supplementary Fig. 10a ). Truncated SHB1 N520 or C325 was fused to YFP C and used in BiFC assays against full-length CCA1 or LHY that was fused to YFP N . The N520:YFP C fusion protein formed fluorescence pairs with either CCA1:YFP N or LHY:YFP N in Nicotiana leaves (Supplementary Fig. 10b ). The C325: YFP C fusion protein that contains the EXS domain did not interact with CCA1:YFP N or LHY:YFP N in the BiFC assays. Both N520:YFP C and C325: YFP C fusion proteins were probed with anti-HA antibodies and expressed at comparable levels (Supplementary Fig. 12a ). CCA1 and LHY are MYB transcription factors and contain a conserved MYB DNA-binding domain at their N termini that is approximately located from amino acids 22–72. We made constructs in which the N-terminal 173 amino acids of CCA1 or LHY were fused to YFP N (N173:YFP N ) or the C-terminal sequence after amino acid 173 was fused to YFP N (CCA1 C435:YFP N or LHY C487:YFP N ) (Supplementary Fig. 11a ). The C terminus but not the N-terminal MYB binding domains of CCA1 or LHY interacted with full-length SHB1 in the BiFC assays (Supplementary Fig. 11b ). Various controls were also included to support the specificity of the interactions. Of the total proteins probed with anti-Myc antibodies, CCA1 or LHY N173:YFP N , CCA1 C435:YFP N and LHY C487:YFP N fusion proteins were expressed at comparable levels (Supplementary Fig. 12b ). CCA1 and LHY co-act with SHB1 SHB1 and CCA1 or LHY were required for PIF4 expression giving that knocking down of SHB1 or knocking out of CCA1 / LHY reduced PIF4 expression (Fig. 1a, e ). We conducted in vivo trans-activation experiments in Arabidopsis cca1 lhy protoplasts with various constructs (Fig. 6d ). We used a PIF4 promoter::LUC reporter along with a CaMV 35 S::REN residing on the same vector to control differences in transformation efficiency. We delivered CCA1 and LHY driven by their native promoter and SHB1 driven by 35 S promoter as effectors to cca1 lhy (Fig. 6d ). We used the 35 S promoter for SHB1 giving that its native promoter drives a very low level of expression and SHB1 is not rhythmically expressed (Supplementary Fig. 1c ). Compared with controls without any effector proteins delivered, delivery of the pCCA1::CCA1:MYC or pLHY::LHY:MYC construct alone to cca1 lhy barely activated the expression of LUC from the PIF4 promoter either in the dark or under red light (Fig. 6e ). Delivery of the 35 S::SHB1:MYC construct alone to cca1 lhy also exhibited minimal effects on the transcription of LUC from the PIF4 promoter. When pCCA1::CCA1:MYC and 35 S::SHB1:MYC were codelivered to cca1 lhy , the transcription of LUC from the PIF4 promoter was activated weakly in the dark but strongly under red light (Fig. 6e ). The effects on LUC transcription from the PIF4 promoter were considerably less dramatic when 35 S::SHB1:MYC was codelivered with pLHY::LHY:MYC either in the dark or under red light. CCA1 protein levels were comparable to that of LHY protein (Supplementary Fig. 12c ). CCA1 or LHY likely recruits SHB1 to the PIF4 promoter, and SHB1 mediates red light-induced PIF4 expression. This red light induction was blocked in phyB-9 under red light (Fig. 6f ). The levels of SHB1, CCA1, and LHY proteins were not different between transformed protoplasts maintained in the dark or under red light (Supplementary Fig. 12c ). The nuclear localization of SHB1:GFP was not affected in the dark compared with that under red light (Supplementary Fig. 12d ). Light and temperature are two important environmental signals that regulate plant growth and development. However, excess light often damages the photosynthetic apparatus and frequently causes photoinhibition. Plants thus evolve a series of strategies to achieve optimum photomorphogenesis. Here we demonstrate a regulatory desensitization step involving SHB1, CCA1/LHY, and PIF4. We proposed a model explaining how CCA1/LHY and SHB1 upregulate PIF4 expression (Fig. 6g ). Our study suggests that the highly expressed circadian clock proteins CCA1 and LHY in the morning recruits SHB1 to activate red light-induced PIF4 expression and desensitize light responses. PIF4 is also a positive regulator of thermomorphogenesis. When temperature increases after morning, the interaction of SHB1 with CCA1 may sustain PIF4 expression to allow plants to better adapt to the temperature-increasing environment. Alternatively, PIF4 transcription allows plants to monitor day-time shade and temperature, which eventually influences PIF4 protein accumulation and activity. The EC formed by LUX, ELF3, and ELF4 proteins peaks at dusk, binds to the PIF4 promoter via the LUX transcription factor, and represses PIF4 transcription in the early evening [46] . EC may recognize two binding elements near the CCA1 and LHY-binding elements. The occupation of the elements by EC and possibly PRRs in the dark may interfere with the binding of CCA1 and LHY to the PIF4 promoter. Indeed, CCA1 and LHY were not associated with the PIF4 promoter in the dark (Fig. 4c and Supplementary Fig. 4c ). Near dawn, CCA1 and LHY associate with the PIF4 promoter, recruit SHB1 to activate PIF4 transcription and promote growth, such as hypocotyl elongation (Fig. 6g ). CCA1 was originally discovered as an activator of a dawn gene LHCB [12] . CCA1 and LHY also repress the evening element-containing genes at dawn [49] . We discovered a new role of CCA1 and LHY to directly recruit SHB1 that mediates red light-induced expression of PIF4 in the morning and thereafter. As such, PIF4 transcription peaks after the middle of the day. ChIP-seq analysis identified the regions of CCA1 occupancy at many EE-containing, evening-expressed, clock-regulated genes in the Arabidopsis genome [48] . CCA1 recognition elements are also located near many genes with peak expression in the morning and in proximity to genes that do not cycle in LL conditions. CCA1 recognizes the canonical EE (AAATATCT) in LL conditions, and the binding capacity of CCA1 is more affected by alteration in the TCT sequence compared with alterations in the ATA or AA [50] . In our yeast one-hybrid analysis, CCA1 only recognizes the M1 element sequence ATATCT, not the M2 element sequence ATATCA in the PIF4 promoter (Fig. 5a, c and Supplementary Fig. 6 ). The last base in the core sequence is apparently critical for CCA1 recognition. In addition, the flanking sequences may also affect the affinity of CCA1 to its binding elements. PIFs belong to a large family of basic helix-loop-helix (bHLH) proteins and exhibit a variety of different functions [51] . Monogenic pif3 , pif4 , pif5, and pif7 null mutants exhibit light-hypersensitive seedling phenotypes, whereas PIF4 , PIF5, and PIF7 are clock regulated [8] , [52] . The three PIFs promote the elongation of hypocotyls and petioles during vegetative growth in a redundant manner [39] , [53] , [54] , [55] . PIF4 has a more-prominent role than PIF5 [56] , [57] . Among the PIF genes, SHB1 specifically regulates the red light-induced expression of PIF4 and likely PIF7 (Fig. 1a and Supplementary Fig. 1a ). Light-activated phyB interacts with PIF4 and targets it for post-transcriptional degradation following the entire light period [53] , [58] , [59] . In these experiments, a CaMV 35 S promoter-driven PIF4 construct was used. On the other hand, PIF4 reaccumulates after a few hours of light treatment [60] , [61] . When PIF4 was driven by its native promoter in a recent study, PIF4 protein accumulated in the light period from ZT0 to ZT8 but not in the dark period from ZT12 to ZT20 [42] . Despite continuous PIF4 degradation, the upregulation of PIF4 expression by CCA1 and SHB1 throughout the day might be responsible for the reappearance of PIF4 protein, constituting a negative regulatory step to antagonize photomorphogenesis. Plant materials and growth conditions Arabidopsis thaliana ecotype Columbia-0 (Col) and Wassilewskija (Ws) were used as wild-type plants. The mutant lines shb1 , shb1-D, and pif4 were described previously [37] , [53] . cca1–11 , cca1–11 lhy-21, and ELF4:GFP seeds were from Gang Li, and lhy-21 seeds were from ABRC ( https://abrc.osu.edu/ ). The shb1-D pif4 double mutant was generated by crossing shb1-D to pif4 and PCR-genotyped using the primers described previously [37] . shb1 cca1 lhy or shb1-D cca1 lhy triple mutant was generated by crossing shb1 or shb1-D to cca1 lhy double mutant and PCR-genotyped using the primers listed in table S1 . All plants were grown in a growth room with a 16 L/8D cycle at 22 °C for seed propagation. For circadian expression analysis, Arabidopsis seedlings were entrained under a 12-hr white or red light and 12-hr dark cycle for 7 days, and then released to continuous white or red light for the following days as described in the figure legends. Similar results were observed when seedlings were released to continuous white or red light for one day and then sampled for the following days. Quantitative RT-PCR For quantitative reverse transcription-polymerase chain reaction (RT-PCR) analysis, total RNA was extracted from seedlings using the MiniBEST Plant RNA Extraction Kit (Takara) or the SV Total RNA Isolation Kit (Promega). SuperScript™ II Reverse Transcriptase (Invitrogen) was used to synthesize cDNA from the RNA. Quantitative real-time PCR was performed with the TransStart Tip Green qPCR SuperMix (Transgen Biotech) on a QuantStudio™ 6 Flex Real-Time PCR machine. The thermal cycling program was 95 °C for 5 min, followed by 40 cycles of 95 °C for 10 s, 56 °C for 10 s and 72 °C for 20 s. The last step involves a one-cycle dissociation stage at 95 °C for 5 s, 65 °C for 1 min, 98 °C for 1 min and 40 °C for 10 s. Most RT-PCR were performed with three biological replicates unless it is specifically indicated in the figure legends. Each biological replicate was represented by three technical replicates. The expression levels of specific genes were normalized to that of UBQ10 and were presented relative to the expression levels in wild type. 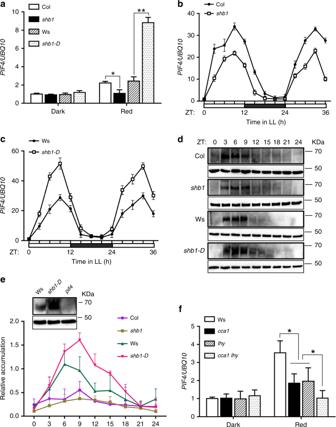Fig. 1 SHB1 and CCA1/LHY regulatePIF4expression under red light.aPIF4expression in 4-day-old Col,shb1, Ws, andshb1-Dseedlings in the dark and under 15 μmol  m−2s−1red light for 3 hr. * and ** indicate significance levelsp< 0.05 andp< 0.01, respectively. ns indicates not significant by Student’s two-tailed heteroscedasticttests in this figure and subsequent figures.PIF4expression in Col andshb1bor Ws andshb1-Dcunder continuous red light after entrained under 12-hr light and 12-hr dark for 7 days from two biological replicates.dPIF4 protein accumulation in Col,shb1, Ws, andshb1-Dunder 12-hr red light and 12-hr dark photoperiod, shown as representative images from three biological replicates.ePIF4 protein quantification normalized to actin with standard error bars. The control blot shows PIF4 accumulation in Ws,shb1-Dandpif4at ZT6.fPIF4expression in Ws,cca1, lhy,andcca1 lhyin the dark and under 15 μmol m−2s−1red light. Expression ofPIF4in each sample was normalized to that ofUBQ10, and data are presented as the means ± SE. Source data are provided as a Source Data file The gene-specific primers for qRT-PCR analysis are listed in Supplementary Table 1 . Hypocotyl length measurement Seeds were sterilized by 1% (v/v) sodium hypochloride and 0.2% (v/v) sodium dodecyl sulphate (SDS) and plated on ½ MS medium. After a 3-day vernalization at 4 °C, seeds were treated with white light for 2–3 h and then incubated under 10 μmol m −2 s −1 red light for 4 days. For thermomorphogenesis, Arabidopsis seedlings were grown under continuous fluorescent white light (30 μmol m −2 s −1 ) at 20 °C for 7 days or at 20 °C for 4 days followed by growth at 29 °C for 3 days. More than 50 seedlings were photoimaged and hypocotyl lengths were measured using ImageJ software ( http://rsb.info.nih.gov/ij ). Hypocotyl experiments were repeated thrice, and one representative dataset was shown. About 50 seedlings were measured for each genotype. For PIF4 expression analysis at 29 °C, seedlings were grown at 20 °C for 5 days and then incubated at either 20 °C or 29 °C for 4 hr before total RNA was extracted. Plasmid construction All primers used to make plasmid constructs were listed in Supplementary Table 1 . All constructs, except for the plasmids used for yeast one-hybrid (Y1H) assay, were made by using the gateway system. In general, the full-length genomic coding region was PCR amplified from Col genomic DNA, cloned into the pCR8/GW/TOPO TA vector, and then recombined into the corresponding destination vectors. To examine the in vivo function of M1 element in PIF4 promoter, a genomic fragment that contains PIF4 promoter up to −1524 bp and coding sequence was cloned into the TA vector. This TA clone was then used as template to mutate the M1 element as base substitution or deletion by a reverse-PCR procedure (TOYOBO, SMK-101). Transgenes were verified by using PIF4-F and c-Myc-R primers. Protein isolation and western blot To detect rhythmic PIF4 accumulation in Col, shb1 , Ws, and shb1-D , seedlings were first grown under 12-hr 2 μmol m −2 s −1 red light and 12-hr dark for 5 days and then sampled at ZT0 and every 3 h thereafter for 24 h. Protein isolation buffer contains 100 m m MOPS pH 7.6, 100 m m NaCl, 10% glycerol, 40 m m 2-mercaptoethanol, 5% SDS, 1× protease inhibitor cocktail from Roche, and 2 m m phenylmethylsulfonyl fluoride (PMSF). Eighty μl buffer were added to 100 μg grinded powder. The mixture was immediately heated at 70 °C for 10 min and separated on 8% SDS–PAGE gel. PIF4 protein was monitored by western blot using anti-PIF4 antibody AS16 3955 (Agrisera, Sweden) from three biological replicates. Protein quantification was performed with IMAGEJ normalized to an actin band. To examine the accumulation of tagged proteins in transgenic plants, the proteins were isolated in buffer that contained 50 m m Tris-HCl pH 8.0, 10 m m EDTA, 1% SDS, 1 m m PMSF and 1× protease inhibitors (Roche). The tagged proteins were detected in western blot using anti-GFP ab1218 (Abcam, Cambridge, MA), anti-FLAG ab49763 (Abcam, Cambridge, MA) and anti-MYC ab32 (Abcam, Cambridge, MA) antibodies. To examine the accumulation of tagged proteins in transient assays, the proteins were isolated in buffer that contained 50 m m Tris-HCl pH 7.5, 150 m m NaCl, 0.1% NP-40, 4 m urea, and 1 m m PMSF. The tagged proteins were detected by anti-HA CW0092 (CWBIO, China) and anti-MYC antibodies as described above. Total proteins in Supplementary Fig. 12c were extracted from protoplasts by boiling in 2× SDS loading buffer at 95 °C for 10 min. The tagged proteins were detected using anti-GFP and anti-MYC antibodies as described above. ChIP assay ChIP assays were performed as described previously [44] , [62] . Seedlings that have 35 S::SHB1:GFP , 35 S::CCA1:FLAG or 35 S::LHY:MYC transgene were grown in the dark or under 15 μmol m −2 s −1 red light for 5 days, and then cross-linked for 30 min in 1% formaldehyde solution under vacuum. For rhythmic ChIP analysis, Col wild type and 35 S::SHB1:GFP transgenic plants were grown under 12-hr red light and 12-hr dark for 3-weeks, and sampled at ZT0 and every 3 h thereafter for 24 h. The plant materials were ground for 10 min on ice in nuclear isolation buffer with 1% formaldehyde, and cross-linking was quenched by adding glycine to a final concentration of 125 m m . The chromatin complex was isolated by nuclear lysis buffer (50 m m Tris-HCl pH 8.0, 10 m m EDTA, 0.5% SDS, 0.1 m m PMSF and 1 × protease inhibitors) and sheared by sonication to generate fragments that were ~ 300–500 bp. The sonicated chromatin complex was then immunoprecipitated by anti-GFP, anti-FLAG, and anti-MYC antibodies as previously described. For rhythmic ChIP analysis, the sonicated chromatin complex was harvested by anti-CCA1 R1234–3 (Abiocode, Agoura Hills, CA), anti-LHY R3095–2 (Abiocode, Agoura Hills, CA) and anti-GFP antibodies. After the reversal of cross-linking, DNA was precipitated in the presence of glycogen (Thermo Fisher) and analyzed by ChIP-qPCR. Most ChIP-PCR were performed with three biological replicates unless it is specifically indicated in the figure legends. Each biological replicate was represented by three technical replicates. The fold enrichment of the specific chromatin fragment was normalized to the UBQ10 amplicon. All primers used for ChIP-qPCR were listed in Supplementary Table 1 . Yeast one-hybrid (Y1H) assay A native 424-bp DNA fragment in the PIF4 promoter was PCR amplified and cloned into the Hind III and Sal I sites of the pAbAi vector (Clontech). Three tandem copies of the putative CCA1/LHY-binding element M1 or M2 were synthesized as oligonucleotides and ligated into the Hind III and Sal I sites of the pAbAi vector (Clontech). Each repeat of the element has a GCTGTA ATATCT TTATGC or TTCCAC ATATCA GGTTAT sequence with a 6-bp flanking sequence on either side of the core elements. The pAbAi vectors harboring the constructs were integrated into the genome of the Y1H Gold yeast strain. The coding sequences of CCA1 and LHY were PCR amplified from cDNA generated from Arabidopsis Col total RNA and cloned into the pGADT7-AD vector (Yeast Protocols Handbook by Clontech, Mountain View, CA). Transformants were selected on minimal synthetic dropout (SD) medium lacking Leu, Trp, and Ura. Yeast cells grown in SD/-Leu/-Trp/-Ura broth were diluted to OD 600 0.5 and plated on SD/-Leu/-Trp/-Ura plate with or without AbA as described by the Matchmaker Gold Yeast One-Hybrid Library Screening System Protocol (Clontech, Mountain View, CA). BiFC assay BiFC experiments were conducted as described [63] . To generate the BiFC constructs, CCA1 or LHY cDNA and SHB1 genomic sequence without their stop codons were PCR amplified and subcloned into the binary vectors pSPYNE and pSPYCE under the control of the cauliflower mosaic virus (CaMV) 35 S promoter. pSPYNE::CCA1 or LHY was co-transformed with pSPYCE::SHB1 into N. benthamiana leaves by agroinfiltration. Their interactions in N. benthamiana leaves were analyzed using an Olympus fluorescence microscope (Olympus BX53 with a DP26 CCD camera) or a confocal microscope (Leica TCS SP5 II). Co-IP assay For co-IP assays, total protein of 35 S::SHB1:GFP and 35 S::CCA1:FALG or 35 S::LHY:MYC seedlings was extracted using IP buffer (10% Glycerol, 25 m m Tris-HCl pH 7.5, 1 m m EDTA, 150 m m NaCl, 0.1% Triton-100, 2 m m β-mercaptoethanol, 1 m m PMSF and 1 × protease inhibitors). After centrifugation at 13,000 rpm for 20 min, the two sources of proteins were mixed and incubated for 2–3 h at 4 °C. 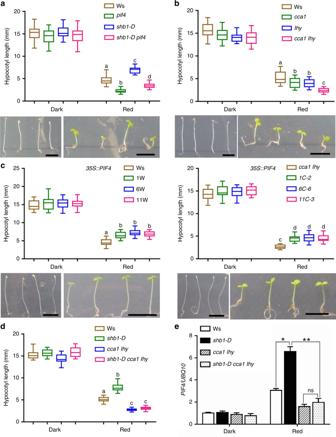Fig. 2 Genetic interaction ofPIF4withSHB1orCCA1/LHY. Hypocotyl lengths of Ws,pif4,shb1-D,andshb1-D pif4a; Ws,cca1,lhy,andcca1 lhyb; three35S::PIF4:GFP(pMDC83) transgenic lines in Ws orcca1 lhyc; and Ws,shb1-D, cca1 lhy,andshb1-D cca1 lhydin the dark or under 10 μmol m−2s−1red light for 4 days. Bar = 5 mm. Box plots display medians as horizontal lines, interquartile ranges as boxes and whiskers extending 1.5 times the interquartile range in this and subsequent figures. Significance levels by Student’s two-tailed heteroscedasticttests in a:p< 0.001 betweenaandb,aandc,aandd,bandd, orcandd; inb:p< 0.01 betweenaandb,p< 0.001 betweenaandcorbandc; inc:p< 0.001 betweenaandborcandd; ind:p< 0.001 betweenaandb,aandcorbandc.ePIF4expression in Ws,shb1-D, cca1 lhy,andshb1-D cca1 lhy.PIF4expression in each sample was normalized to that ofUBQ10, and data are presented as the means ± SE. Source data are provided as a Source Data file The mixture was then incubated with the anti-GFP rabbit polyclonal antibody 10004D (Thermo Fisher, CA) for another 2 h. The beads were washed four times with IP buffer. 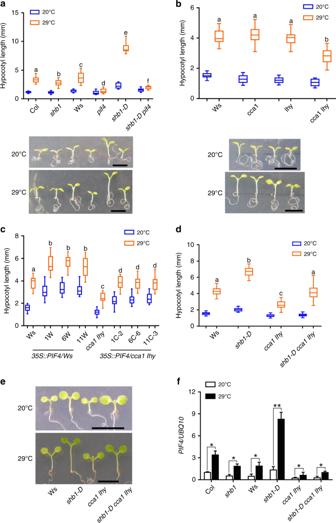Fig. 3 CCA1/LHY and SHB1 enhancePIF4expression and thermomorphogenesis. Hypocotyl lengths of Col,shb1, Ws,pif4,shb1-D, andshb1-D pif4a; Ws,cca1,lhy, andcca1 lhyb; three35S::PIF4:GFPlines in Ws orcca1 lhyc; and Ws,shb1-D,cca1 lhy,andshb1-D cca1 lhyd,eunder 30 μmol m−2s−1white light at 20 °C for 7 days or 20 °C for 4 days followed by 29 °C for 3 days. Bar = 5 mm. Significance levels by Student’s two-tailed heteroscedasticttests in a:p< 0.001 betweenaandb,candd,cande,candf,dande, oreandfandp< 0.01 betweendandf; inb:p< 0.001 betweenaandb; inc:p< 0.001 betweenaandborcandd; ind:p< 0.001 betweenaandb,aandcorbandc.fPIF4expression in Col, shb1, Ws,shb1-D,cca1 lhy,andshb1-D cca1 lhy. Seedlings were grown at 20 °C for 5 days and then incubated at 20 °C or 29 °C for 4 h.PIF4expression in each sample was normalized to that ofUBQ10, and data are presented as the means ± SE. Source data are provided as a Source Data file 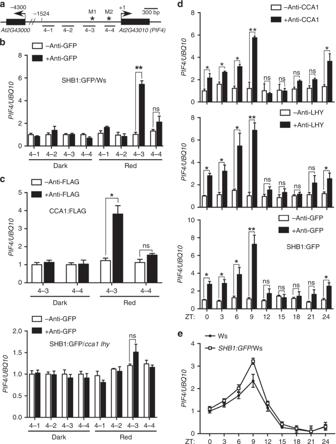Fig. 4 SHB1 and CCA1/LHY are associated with thePIF4promoter.aPIF4promoter demonstrating the chromatin regions (4–1, 4–2, 4–3, and 4–4) used for ChIP-quantitative PCR analysis and the potential Myb-binding sites M1 and M2 (asterisks). Association of SHB1:GFPband CCA1:FLAG or SHB1:GFP incca1 lhycwith thePIF4promoter.dRhythmic association of CCA1, LHY, or SHB1:GFP with thePIF4promoter under 12-hr dark and 12-hr red light cycles from two biological replicates. Enrichment of DNA fragments was quantified by qPCR and normalized to that ofUBQ10.eRhythmicPIF4expression at various ZT points in Ws and35S::SHB1:GFPtransgenic plants under 12-hr dark and 12-hr red light cycles. Data are presented as the means ± SE calculated from two biological replicates. Source data are provided as a Source Data file The pelleted beads were boiled in 60 μl 2 × SDS buffer and separated by 8% SDS–PAGE. Western blots were probed by using anti-FLAG or anti-MYC antibodies at a 1:1000 dilution. Transient trans-activation assay Arabidopsis mesophyll protoplast isolation and transformation were performed as described [64] . pCCA1::CCA1:MYC , pLHY::LHY:MYC and 35 S::SHB1:MYC were used in effector constructs. The pGreen II−0800-LUC vector that bears pPIF4::LUC and 35 S::REN was used as a reporter construct. 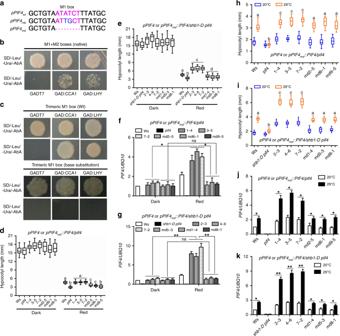Fig. 5 CCA1 and LHY recognize MYB M1 box in thePIF4promoter.aPotential MYB-binding element M1 is noted in red, and the bases mutated are noted in blue. mb and md indicate mutation by base substitution and deletion, respectively. Yeast one-hybrid assays for CCA1 or LHY inpGADT7over a 424-bp fragment that contains both M1 and M2 elements from thePIF4promoter in thepAbAivectorband for CCA1 or LHY inpGADT7over trimeric repeats of wild type (upper) or mutated (lower) M1 elementc. Golden Y1H cells were grown on SD/-Leu/-Ura media with or without 300 ng/ml Aureobasidin A (AbA) selection. Hypocotyl lengths of Ws,pif4andpPIF4orpPIF4md::PIF4inpif4dand Ws,shb1-D pif4andpPIF4orpPIF4md::PIF4inshb1-D pif4e.PIF4expression in Ws,pif4andpPIF4orpPIF4md::PIF4inpif4fand Ws,shb1-D pif4andpPIF4orpPIF4md::PIF4inshb1-D pif4g. The seedlings were grown in the dark or under 10 μmol m−2s−1red light for 4 days. Hypocotyl lengths of Ws,pif4andpPIF4orpPIF4md::PIF4inpif4hand Ws,shb1-D pif4andpPIF4orpPIF4md::PIF4inshb1-D pif4iunder 30 μmol m−2s−1white light at 20 °C for 7 days or 20 °C for 4 days followed by 29 °C for 3 days.PIF4expression in Ws,pif4andpPIF4orpPIF4md::PIF4inpif4jand Ws,shb1-D pif4andpPIF4orpPIF4md::PIF4inshb1-D pif4kgrown at 20 °C for 5 days and then incubated at 20 °C or 29 °C for 4 h. Significance levels by Student’s two-tailed heteroscedasticttests ind:p< 0.001 betweenaandb,p< 0.01 betweenaandc,p< 0.05 betweenbandc; ine:p< 0.001 betweenaandb,aandc,bandcorcandd,p< 0.01 betweenaandd,p< 0.05 betweenbandd; inh:p< 0.001 betweenaandborbandc,p< 0.01 betweenaandc; ini:p< 0.001 betweenaandb,aandcorbandc. Source data are provided as a Source Data file 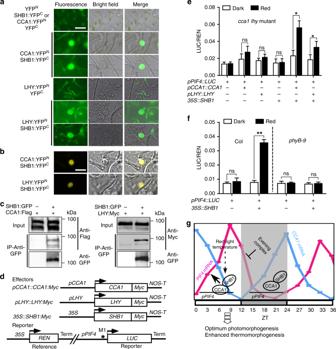Fig. 6 SHB1 co-acts with CCA1 and LHY.aBiFC fluorescent images of YFPNwith SHB1:YFPC, CCA1:YFPNor LHY:YFPNwith YFPC, and CCA1:YFPNor LHY:YFPNwith SHB1:YFPC.bBiFC confocal images of CCA1:YFPNor LHY:YFPNwith SHB1:YFPC. Images were captured 48–72 h inNicotianaleaf epidermal cells after Agrobacteria transfection. Bar = 10 μm.cCo-immunoprecipitation (Co-IP) of CCA1:FLAG or LHY:MYC by SHB1:GFP in protein extracts prepared from transgenicArabidopsiswith anti-GFP antibody.dEffector, reporter, and reference constructs used. Arrowheads indicate transcription start sites, and NOS-T represents polyadenylation signal from the nopaline synthase gene. Asterisk indicates the location of the M1 element in thePIF4promoter. Relative LUC/REN activity incca1 lhytransformed with a reporter along withpCCA1::CCA1:MYC,pLHY::LHY:MYCor35S::SHB1:MYCeand in Col orphyB-9transformed with reporter in the absence or presence of35S::SHB1:MYCfin the dark or under red light. Source data are provided as a Source Data file.gA model explaining the regulation of CCA1 or LHY and SHB1 overPIF4expression.PIF4expression is repressed by the evening complex (EC) or PRRs at early evening. Toward the end of night and after dawn, CCA1 recruits SHB1 to mediate red light induction ofPIF4expression. This constitutes a signaling loop to optimize photomorphogenesis and enhance thermomorphogenesis Luciferase activity was measured using the Dual-Luciferase Reporter Assay System (Promega, USA). Relative luciferase activity was normalized to REN activity as a LUC/REN ratio for each biological sample. Experiments were repeated thrice and each biological replicate was represented by three technical replicates.